Stirring competes with chemical induction in chiral selection of soft matter aggregates Chirality, the absence of mirror symmetry, can be equally invoked in relation to physical forces and chemical induction processes, yet a competition between these two types of influence is rarely reported. Here we present a self-assembled soft matter system in which chiral selection is controlled by the combined independent action of a chiral dopant and vortical stirring, which are arbitrarily coupled, either constructively or destructively. In the latter case, perfect compensation, that is, absence of a net chiral effect, is realized. The induced enantiomorphic excess is measured in terms of the statistical imbalance of an ensemble of submillimetre domains, where achiral molecules self-assemble with a well-defined orientational chirality that is unambiguously resolved using optical microscopy. The possibility of combining top-down and bottom-up strategies to induce a chiral predominance in a supramolecular system of achiral components should be recognized as a new twist in the process of chiral recognition, selection and control. Chirality is a pervasive dissymmetry, as defined by Pasteur, and a fundamental constraint in nature [1] , [2] . In particular, one anticipates that achiral substances can be transformed, at most, into a racemic mixture of equally represented enantiomers, or into an enantiopure system with equal probability for the two enantiomers. Apart from the handedness imparted by proto-chiral organizing surfaces [3] , oriented reacting interfaces [4] , and aligning [5] or confining [6] boundaries, the balance above may be broken under the intervention of one within a few physical forces of signed helicity [7] , [8] , or through the effect of a chiral chemical modifier. In general terms, there is still the pending issue of whether a chiral physical force may be opposed in an effective way to a chiral chemical intervention. As a matter of fact, if we all recognize that there is no fundamental difference between 'physical' and 'chemical' handedness, we must admit that physical forces and chemical induction processes have rarely been directly confronted in terms of their respective potential chiral strengths. In soft matter-oriented research, control of imparted chirality is particularly valuable, both from a fundamental as well as an applied perspective [9] , [10] . A chiral modifier, chemically compatible with the host system, is often employed to imprint an achiral mesophase with a well-defined handedness [11] . For instance, on using a chiral mesogenic molecule as a dopant, a nematic liquid crystal phase will convert into a chiral nematic or cholesteric phase, in which the average molecular orientation develops a spatially organized helical arrangement, with a characteristic pitch and twist sign, which depend on subtle non-covalent interactions between the modifier and the host system [12] . For a given dopant concentration, this effect is maximized when only one of the enantiomers is present, and it vanishes when the dopant consists of a racemic mixture. On the other hand, a chiral imbalance can be imparted to certain systems composed of achiral molecules or to racemic mixtures of two enantiomers by means of a suitable macroscopic chiral force, such as circularly polarized light. For instance, the latter permits the interconversion of enantiomers in a racemic photoresponsive material [13] , or provides a way for chiral induction on achiral azobenzene-based liquid crystalline polymer films [14] , [15] and, more recently, has rendered possible a strategy for chiral induction on domains of achiral bent-shape dimers [16] . In a different context, another procedure consists in using unpolarized light in the presence of a coaxial magnetic field [17] . Differently from electromagnetic interventions, we will focus here on chiral selection by vortical shearing [2] . While this triad involves forces of physical character, we may qualify the above-referred induction by a chiral modifier as a manifestation of a genuine chemical effect. Focusing on hydrodynamic effects [18] , [19] , [20] , the relationship between stirring and material-based chirality traces back to the observation of the single mirror-image crystallization of sodium chlorate from a solution of no handedness solute [21] . More striking is the report that the combination of soft aggregation and stirring may lead not only to chiral induction [22] , [23] but, more importantly, also to sign selection, in both three [24] , [25] and two dimensions [26] , [27] . Discussions on the true nature of such an enantioselection in three-dimensional aggregates have raised some controversy [28] , [29] , [30] , [31] , [32] , [33] . Recently, d'Urso et al . [34] have hinted at the possibility to exert enantioselective control on the supramolecular assembly of achiral components doped with a chiral complex by means of vortex flow. However, their system does not allow obtaining conclusive results, as a hypothetical genuine chiral effect cannot be decoupled from a transient fibre-alignment mechanism. Here we present the realization of the unambiguous coupling between a signed chiral force (vortex flow) and an intrinsically chiral chemical system during enantioselective control in monomolecular films of amphiphilic molecules self-assembled at the air/water interface. We demonstrate that physical, down-scale and chemical, up-scale, chiral influences can meet midway and their responses be arbitrarily opposed or enhanced. Characterization of the chirally resolved Langmuir monolayer The emergence of chiral structures is documented in insoluble monolayers at the air/water interface (Langmuir monolayer), both involving chiral [35] and non-chiral components [36] , [37] . Here we work with an azobenzene-based photoresponsive achiral amphiphile, Azo1 (see Methods ), known to feature spontaneous chiral resolution. We disperse Langmuir monolayers with a nearly pure composition of the cis isomer, and let the system relax at constant temperature and spreading area under room light conditions. Upon spontaneous transformation into the trans isomer, phase separation of the two isomeric forms leads to the formation of a two-dimensional emulsion in which submillimetre circular mesophase discs, rich in the trans isomer, are surrounded by an isotropic continuous cis phase ( Fig. 1 ). Using polarizing reflection microscopy at the Brewster angle (BAM), we are able to detect that, inside these discs, surfactant molecules in the trans configuration organize with a uniform tilt with respect to the surface normal, and a spatially varying in-plane projection, which can be characterized by a two-dimensional vector field, c ( x , y ). Reflectivity patterns inside the discs unambiguously reveal that, on average, molecules are locally tilted along a direction parallel to the domain boundary (bend-like ordering) [37] , either clockwise (CW) or counter-clockwise (CCW), that is, c =± r × τ , where r is the radial coordinate with respect to the domain centre, τ is the unit vector normal to the air/water interface and ' × ' denotes the vector product. This defines the two enantiomorphic configurations of the orientational order that are equally represented in the absence of any chiral influence ( Fig. 1 ). 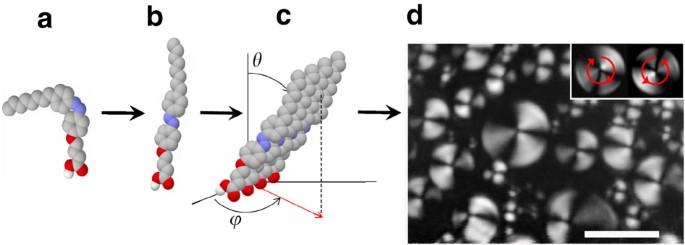Figure 1:Self-assembly leading to the formation of a two-dimensional emulsion featuring chirally resolved domains. Transazobenzene surfactant molecules (b), resulting from the spontaneous isomerization of thecisisomer (a), self-assemble at the air/water interface into segregated chirally resolved circular domains surrounded by thecis-rich matrix (d). Long-range orientational order inside the domains is characterized using BAM imaging (d) in terms of a constant tilt angle,θ, and a spatially varying azimuth,, (c) which defines an orientational handedness for each domain. Insets in the grayscale BAM image illustrate the field lines, tangential to the local molecular orientation, for the two enantiomorphic circular domains. The line segment is 100 μm long. The orientation of the three dark brushes in the BAM image of a given domain allows identifying its handedness. Inspection of an extended region of the monolayer (several square centimeters) reveals, in the absence of any chiral influence, an equal presence of domains of both handednesses. Figure 1: Self-assembly leading to the formation of a two-dimensional emulsion featuring chirally resolved domains. Trans azobenzene surfactant molecules ( b ), resulting from the spontaneous isomerization of the cis isomer ( a ), self-assemble at the air/water interface into segregated chirally resolved circular domains surrounded by the cis -rich matrix ( d ). Long-range orientational order inside the domains is characterized using BAM imaging ( d ) in terms of a constant tilt angle, θ , and a spatially varying azimuth, , ( c ) which defines an orientational handedness for each domain. Insets in the grayscale BAM image illustrate the field lines, tangential to the local molecular orientation, for the two enantiomorphic circular domains. The line segment is 100 μm long. The orientation of the three dark brushes in the BAM image of a given domain allows identifying its handedness. Inspection of an extended region of the monolayer (several square centimeters) reveals, in the absence of any chiral influence, an equal presence of domains of both handednesses. Full size image Chiral selection Uncompensated handedness appears when we add a small amount of a chiral surfactant modifier (Azo-R or Azo-S, see Methods ) to the Azo1 spreading solution, before dispersion. The signature of a chiral dominance manifests itself as a different amount of CW versus CCW bend-like domains. In quantitative terms, such a difference, normalized by the total number of counted domains, defines an enantiomorphic excess of CW domains ( ee CW ). In our case, 6% of R -enantiomer doping leads to a robust CCW excess, ee CW =−0.54±0.05, which is exactly opposite, within experimental error, to the result for the same amount of the S-form. To evidence the effect of vortical shearing, we now proceed by spreading the monolayer while gently stirring the aqueous subphase (see Methods ). Results plotted versus the signed stirring rate (CW is arbitrarily taken as positive) are summarized in Fig. 2 . For the sake of comparison we include results of the stirred monolayer under racemic conditions, that is, with the same amount of total doping equally distributed among the R and S forms of the chiral modifier. 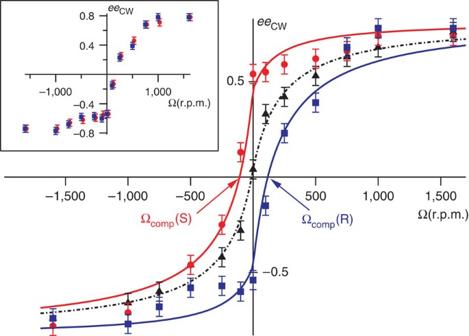Figure 2:Coupling between the chiral modifier and the vortical flow. Enantiomorphic excess,, quantifying the statistical bias of CW bend-like domains as a function of the vortical stirring rate in the presence of different enantiomeric compositions of the chiral dopant: 6% of S-enantiomer (red circles), 6% of R-enantiomer (blue squares) and racemic mixture (3+3%) of R and S enantiomers (black triangles). Error bars correspond to 5% of the full-scale value ofeeCW. Solid lines are a fit to the function, according to the model proposed in the text. Fitted parameters areλ=0.83±0.08,. for enantiomer R, whereas. anda=190±50 r.p.m. for enantiomer S. A similar fit is performed for the racemic mixture, resulting inλ=0.80±0.04,. anda=230±40 r.p.m. In the inset,data for the R-enantiomer are plotted along withfor the S-enantiomer, empirically showing the congruent asymmetry between the effect of the two enantiomers. Figure 2: Coupling between the chiral modifier and the vortical flow. Enantiomorphic excess, , quantifying the statistical bias of CW bend-like domains as a function of the vortical stirring rate in the presence of different enantiomeric compositions of the chiral dopant: 6% of S-enantiomer (red circles), 6% of R-enantiomer (blue squares) and racemic mixture (3+3%) of R and S enantiomers (black triangles). Error bars correspond to 5% of the full-scale value of ee CW . Solid lines are a fit to the function , according to the model proposed in the text. Fitted parameters are λ =0.83±0.08, . for enantiomer R, whereas . and a =190±50 r.p.m. for enantiomer S. A similar fit is performed for the racemic mixture, resulting in λ =0.80±0.04, . and a =230±40 r.p.m. In the inset, data for the R-enantiomer are plotted along with for the S-enantiomer, empirically showing the congruent asymmetry between the effect of the two enantiomers. Full size image The data in Fig. 2 constitute the key result of this work unveiling the concept of chiral coupling from disparate origins. More specifically, they certify the possibility of exact compensation between a chemical chiral influence and an opposing vortical shear. At an equal concentration (6% by weight) of either enantiomer, the compensation stirring rate exhibits the required symmetry . Notice also the apparent dominance of the chiral stirring force against the influence of the chemical dopant, at least in the experiments reported here. Actually, the data series for the three compositions of the chiral dopant converge for absolute values of Ω above 1,000 r.p.m. Finally, the robustness of the phenomenon is clearly evidenced by the perfectly symmetric racemic data , and by the congruent asymmetry of the data series for the two enantiomers (see the inset in Fig. 2 ). Self-assembly of primordial aggregates BAM imaging ( Fig. 3 ) reveals that trans molecules arising from the spontaneous isomerization of the cis azobenzene assemble into elongated primordial aggregates in which c ( x , y ) has a dipolar order with elongated (head–tail asymmetric) molecules featuring an average orientation along the longest dimension. The shape and inner configuration of these aggregates depend on the enantiomeric excess of the chiral dopant: while they are elliptical in shape for a racemic mixture of the chiral dopant, they acquire a bean-like shape for an imbalance of one of the enantiomers. The final chirally resolved circular domains arise from the spontaneous coalescence of primordial elongated domains. Indeed, line tension at the boundary with the cis phase prompts the spontaneous merging of a pair of aggregates with antiparallel polarity, resulting in the formation of a circular domain whose orientational chirality corresponds to that of the dimer formed by the two parent aggregates. Although circular domains of both chiralities are always formed, doping with opposite enantiomers introduces opposite imbalances in their enantiomorphic excess. 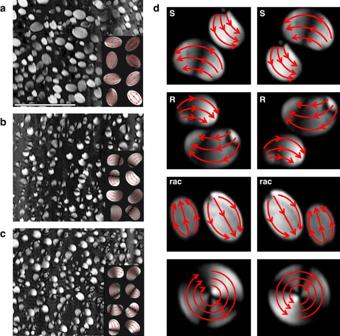Figure 3:Primordial aggregates and formation of bend-like domains. (a–c) BAM micrographs of monolayers featuring self-assembled primordial aggregates under different composition of chiral dopant: racemic dopant mixture with 3% w/w of Azo-S and 3% w/w of Azo-R (a); 6% w/w of Azo-S (b); and 6% w/w of Azo-R (c). As a guide for the eye, a sketch with the approximate BAM image and corresponding estimated field lines for different orientation of the aggregates is shown as an inset in each panel. The line segment in (a) is 500 μm long. A racemic mixture of dopants (a) leads to the self-assembly of achiral elliptical aggregates, whereas in the presence of a chiral dopant (b,c), self-assembled bean-shaped primordial aggregates feature enantiomorphic configurations with complete resolution for the R and S enantiomers. (d) For all dopant composition, the spontaneous coalescence of antiparallel elongated aggregates proceeds through an intermediate dimer-like arrangement and finally results in the formation of enantiomorphic circular bend-like domains. Their orientational chirality (CW for the left column, CCW for the right column) is determined by the handedness of the dimer configuration of the two parent aggregates. The width of each BAM micrograph is 190 μm. Approximate field lines giving the local in-plane molecular orientation are overlaid to each BAM image. Figure 3: Primordial aggregates and formation of bend-like domains. ( a – c ) BAM micrographs of monolayers featuring self-assembled primordial aggregates under different composition of chiral dopant: racemic dopant mixture with 3% w/w of Azo-S and 3% w/w of Azo-R ( a ); 6% w/w of Azo-S ( b ); and 6% w/w of Azo-R ( c ). As a guide for the eye, a sketch with the approximate BAM image and corresponding estimated field lines for different orientation of the aggregates is shown as an inset in each panel. The line segment in ( a ) is 500 μm long. A racemic mixture of dopants ( a ) leads to the self-assembly of achiral elliptical aggregates, whereas in the presence of a chiral dopant ( b , c ), self-assembled bean-shaped primordial aggregates feature enantiomorphic configurations with complete resolution for the R and S enantiomers. ( d ) For all dopant composition, the spontaneous coalescence of antiparallel elongated aggregates proceeds through an intermediate dimer-like arrangement and finally results in the formation of enantiomorphic circular bend-like domains. Their orientational chirality (CW for the left column, CCW for the right column) is determined by the handedness of the dimer configuration of the two parent aggregates. The width of each BAM micrograph is 190 μm. Approximate field lines giving the local in-plane molecular orientation are overlaid to each BAM image. Full size image We propose that the two complementary coalescence events leading to circular domains are kinetically biased due to the asymmetric shape of the parent aggregates ( Fig. 3 ). A similar bias can be introduced by vortical shearing, as the dipolar nature of c ( x , y ) makes the two complementary coalescence events non-equivalent in the presence of stirring. We will introduce a mechanism to explain the reported phenomenon by invoking kinetic arguments that translate into a chemical-kinetics-like model ( Fig. 4 ). The mechanism assumes parallel pathways for the irreversible evolution of the dispersed monolayer under the influence of the dopant and the vortical force. In essence, each pathway is built from three consecutive steps that connect the transformed original cis material into the final trans -rich circular domains. The first step is the nucleation and growth of bean-like elongated primordial aggregates, denoted B , following the spontaneous cis – trans isomerization. The next step involves the formation of the dimer entities with CW and CCW antiparallel dipolar arrangement, which we denote D CW and D CCW . To simplify the notation, let us consider the case of the coupling between vortical flow and doping with the Azo-R enantiomer. An equivalent analysis could be performed with the Azo-S enantiomer. 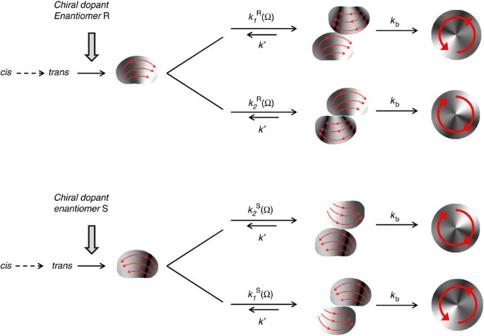Figure 4:Scheme of the kinetic model for chiral selection. Followingcis–transisomerization, bean-shapedtransaggregates nucleate and grow under the chiral influence of the dopant enantiomer. Two distinct parallel pathways, corresponding to the pair of enantiomorphically different dimer configurations, are possible for each dopant enantiomer. We propose that the kinetics of formation of the dimers is described by stirring-dependent rate constants. A final step, which corresponds to the irreversible relaxation of the dimer entity towards the corresponding circular bend-like domain, has a large rate constant,kb. In this scheme, subindices '1' and '2' refer to pathways leading to CCW and CW domains, respectively. Experimental results reported inFig. 2indicate that the presence of chiral dopant favours the pathway involving dimers of bean-shaped domains that face their convex sides. These relationships are correctly captured by the fit of the proposed model to the experimental data.Figure 2indicates that, contrarily, coupling with the flow is enhanced when bean-shaped domains face their flattened sides. This corresponds to the regime where stirring opposes the effect of the chiral dopant. Figure 4: Scheme of the kinetic model for chiral selection. Following cis – trans isomerization, bean-shaped trans aggregates nucleate and grow under the chiral influence of the dopant enantiomer. Two distinct parallel pathways, corresponding to the pair of enantiomorphically different dimer configurations, are possible for each dopant enantiomer. We propose that the kinetics of formation of the dimers is described by stirring-dependent rate constants. A final step, which corresponds to the irreversible relaxation of the dimer entity towards the corresponding circular bend-like domain, has a large rate constant, k b . In this scheme, subindices '1' and '2' refer to pathways leading to CCW and CW domains, respectively. Experimental results reported in Fig. 2 indicate that the presence of chiral dopant favours the pathway involving dimers of bean-shaped domains that face their convex sides. These relationships are correctly captured by the fit of the proposed model to the experimental data. Figure 2 indicates that, contrarily, coupling with the flow is enhanced when bean-shaped domains face their flattened sides. This corresponds to the regime where stirring opposes the effect of the chiral dopant. Full size image We formulate the corresponding model by considering the kinetics of formation of the dimer entities to be described by stirring-dependent rate constants k 1 R (Ω)= k 1 + k 1 st (Ω) for D CCW , and k 2 R (Ω)= k 2 + k 2 st (Ω) for D CW . Here, k 1 st (Ω) and k 2 st (Ω), which vanish under quiescent (no flow) conditions, correspond to the hydrodynamic influence in the chiral selection process, and k 1 = k 1 R (0) and k 2 = k 2 R (0) correspond to the chemical influence due to the presence of a chiral dopant. The dimers will irreversibly coalesce and relax to the corresponding circular domain with a rate constant k b , which we will consider identical for all pathways, as its value is dictated by the rate of relaxation of the molecular orientation inside the fused domains. The two backward kinetic constants, assumed equal to k ′ (see Fig. 4 ), account for the eventual decomposition of the dimers. They are assumed to be significantly lower than their forward counterparts, as once two bean-like domains have contacted they cannot be easily separated again. We apply the quasi steady-state approximation to the concentration of dimer entities, namely, where we have considered a second-order process leading to the formation of the dimer entities through the coalescence of two elongated aggregates. We can thus express ee CW as In this expression, λ is a parameter, 0< λ <1, accounting for the loss of circular bend-like domains due to the different processes involved in the evolution of the monolayer, such as the coalescence of CW and CCW domains, the absorption of bend domains by larger non-circular domains and so on. As an ansatz for the stirring-rate dependence of the rate constants, we propose a linear relationship of the form and , where γ is a proportionality constant and θ( Ω) is the Heaviside function, equal to 1 for CW (Ω>0) and 0 for CCW (Ω<0) stirring, according to the sign prescription adopted in Fig. 2 . These expressions capture the experimental result that the formation of D CW is only favoured by CW stirring, whereas the formation of D CCW is only favoured by CCW stirring. The final expression for ee CW is where we have defined As shown in Fig. 2 , this model provides a good fit for our ee CW experimental values. Symmetry considerations require that the values for the quiescent (Ω=0) kinetic constants are interchanged in the presence of each enantiomer, that is, k 1 R (0)= k 2 S (0), and k 2 R (0)= k 1 S (0). As a result, the influence of each enantiomer is captured by Ω comp , which should have an opposite value for Azo-R and Azo-S, whereas a should be equal for both. The fitted values for these parameters satisfy these symmetry arguments. In fact, the values of Ω comp and a allow to compare the kinetic constants in a quiescent system in the presence of each chiral dopant: for enantiomer R, which favours CCW domains, k 1 ≈3.6 k 2 , and for enantiomer S, which favours CW domains, k 2 ≈3.6 k 1 . This result can be understood from the asymmetric shape of the self-assembled elongated primordial aggregates that makes the coalescence of quasi-antiparallel dimers more likely, from a geometrical point of view, when they face their convex sides than when they face their flattened concave sides. This provides a kinetic advantage for the formation of CCW and CW bend-like domains for the R and S enantiomers, respectively. As a conclusion, the principle of chiral superposition from two independent sources has been unambiguously reported, mechanistically interpreted and modelled here on a simple basis. The realization of such chiral 'algebra' is even more rewarding given the disparate nature of the involved influences: a three-dimensional force of physical nature, operating in centimetre-length scales, facing the chemical effect of a supramolecular level modifier. Notice that this finding is entirely different from previous successful attempts to photomodulate chiral modifier-based influences in doped ferroelectric [38] or cholesteric liquid crystals [39] , or to modify the helicoidal structure of cholesteric liquid crystals by means of an achiral external mechanical field [40] . Unveiled as a new dynamical scenario of chirality control, our contribution should also be envisaged, upon transference of the monolayer into a solid support, as a new strategy for stereocontrol of chemical reactions and responses at chiral surfaces [41] , [42] . Materials We prepare Langmuir monolayers by spreading a chloroform (Baker, p.a.) solution (1 mM) of the surfactant 4-[4-[(4-octylphenyl)azo]-phenoxy] butanoic acid [37] (Azo1) that contains a 6% w/w of the chiral modifier [(S/R)−(+/−)-4-[4-[4-(1-methylheptyloxyphenyl)azo] phenoxy] butanoic acid] (Azo-S, Azo-R), either as pure S/R-enantiomers or as a racemic mixture of the two enantiomers. All surfactants were custom synthesized. 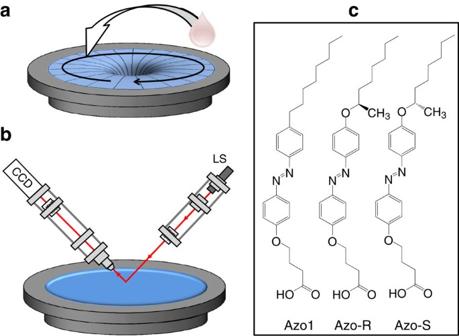Figure 5:Stirred monolayers of surfactant molecules. (a) A single drop of chloroform surfactant solution is deposited at the outer edge of the steady-state funnel generated by a rotating magnetic bar, and is left to evolve under constant stirring for a period of time. (b) The resulting distribution of chiral submillimetre circular monolayer domains is analysed following the arrest of stirring by means of BAM microscopy. The structure of thetransisomer of the three azobenzene surfactant molecules is shown in (c). See Figure 5 for a sketch of the three molecules. Earlier work with Langmuir monolayers of Azo1 [37] revealed that the cis and trans isomers of this surfactant phase separate when spread at the air/water interface. The relative composition of cis and trans isomer can be adjusted by exposing the spreading solution to light of a suitable wavelength. Figure 5: Stirred monolayers of surfactant molecules. ( a ) A single drop of chloroform surfactant solution is deposited at the outer edge of the steady-state funnel generated by a rotating magnetic bar, and is left to evolve under constant stirring for a period of time. ( b ) The resulting distribution of chiral submillimetre circular monolayer domains is analysed following the arrest of stirring by means of BAM microscopy. The structure of the trans isomer of the three azobenzene surfactant molecules is shown in ( c ). Full size image Experimental apparatus The experimental setup consists of a thermostatic black Delrin (polyoxymethilene) circular trough (6 cm diameter, 1.7 cm depth) filled with Milli-Q water ( Fig. 5 ). Before monolayer spreading, a steady-state vortex flow is created in the subphase by means of a reversible magnetic stirrer (J.P. Selecta, Spain) with a submerged cylindrical Teflon-coated magnetic bar (8 mm long, 3 mm diameter). The spreading solution is irradiated with UV light for 10 min to ensure the maximum presence of the cis isomer (97%). Monolayers are subsequently prepared by carefully depositing at the air/water interface one drop (2 μl) of the chloroform surfactant solution at the outer part of the vortical funnel when the subphase is stirred at a constant rate Ω (0<Ω<1,600 r.p.m.). Experiments are conducted at 20 °C with a surface pressure below 1 mN m −1 . Stirring is applied for 35 min under room light. These are the optimal experimental conditions that enhance the competition between the stirring and the chiral modifier. Spontaneous cis to trans isomerization leads to the formation of isolated submillimetre-elongated trans -rich aggregates that coalesce into circular domains with long-range order in the orientation of hydrophobic tails of Azo1 surfactant molecules. Data acquisition and analysis After stopping stirring, we perform a statistical analysis of the population of circular domains of either handedness, which yields the enantiomeric excess parameter. BAM images of the monolayer are recorded using a custom-built instrument, with the analyser set at 60° CCW with respect to the plane of incidence, which contains the y -axis of the images. With this configuration, the orientational handedness of individual circular domains can be unambiguously determined. The microscope is equipped with an XY translation stage to be able to scan the air/water interface. This enables us to obtain data for an extended region of the monolayer (several square centimeters). Exploration is continued during 30 min after stirring is stopped. Simultaneous recording while stirring is unpractical due to the curvature of the interface, as BAM imaging demands a flat interface. BAM images are enhanced and analysed by means of the software ImageJ [43] . How to cite this article: Petit-Garrido, N. et al . Stirring competes with chemical induction in chiral selection of soft matter aggregates. Nat. Commun. 3:1001 doi: 10.1038/ncomms1987 (2012).